Coherent Stern–Gerlach momentum splitting on an atom chip In the Stern–Gerlach effect, a magnetic field gradient splits particles into spatially separated paths according to their spin projection. The idea of exploiting this effect for creating coherent momentum superpositions for matter-wave interferometry appeared shortly after its discovery, almost a century ago, but was judged to be far beyond practical reach. Here we demonstrate a viable version of this idea. Our scheme uses pulsed magnetic field gradients, generated by currents in an atom chip wire, and radio-frequency Rabi transitions between Zeeman sublevels. We transform an atomic Bose–Einstein condensate into a superposition of spatially separated propagating wavepackets and observe spatial interference fringes with a measurable phase repeatability. The method is versatile in its range of momentum transfer and the different available splitting geometries. These features make our method a good candidate for supporting a variety of future applications and fundamental studies. The development of atom interferometry over the last two decades has given rise to new insights into the tenets of quantum mechanics [1] as well as to ultra-high accuracy sensors for fundamental physics [2] , [3] , [4] and technological applications [5] , [6] . Examples range from the creation of momentum state superpositions by accurate momentum transfer of laser photons [7] , [8] allowing high precision measurements of rotation, acceleration and gravity [5] , [6] , [9] , [10] , to the splitting of trapped ultracold atoms by local potential barriers [11] , [12] , [13] allowing the investigation of fundamental properties of quantum systems of a few or many particles, such as decoherence and entanglement [14] , [15] , [16] . One of the tools for atom interferometry is the atom chip [17] , [18] , [19] . The high level of spatial and temporal control of local fields which is facilitated by the atom chip has made it an ideal tool for the splitting of a Bose–Einstein condensate (BEC) into a double-well potential by a combination of static magnetic fields with radio-frequency (RF) [12] or microwave [13] fields. Pure static fields [20] or light fields [21] , [22] have also been used. However, practical atom chip schemes for interferometry with a wide dynamic range and versatile geometries are still very much sought after [23] , [24] , [25] , [26] , [27] , [28] . Such schemes may enable, for example, sensitive probing of classical or quantum properties of solid-state nanoscale devices and surface physics (for example, refs 29 , 30 , 31 , 32 , 33 ). This is expected to enhance considerably the power of non-interferometric measurements with ultracold atoms on a chip, which have already contributed, for example, to the study of long-range order of current fluctuations in thin films [34] , the Casimir–Polder force [35] , [36] , [37] , [38] and Johnson noise from a surface [39] . In addition, interferometry integrated on a chip is a crucial step towards the development of miniature rotation, acceleration and gravitational sensors based on guided matter waves [23] , [27] . One of the earliest attempts to envision atom interferometry was considered shortly after the discovery of the Stern–Gerlach (SG) effect almost a century ago [40] . The SG effect, which has become a paradigm of quantum mechanics [41] , uses a magnetic gradient to split particles into momentum states with different spin projections. SG interferometry was generally judged to be impractical because of the extreme accuracy that would be required, where fundamental issues of phase dispersion stemming from the uncertainty principle were raised (Briegel et al . [42] and references therein), and finally coined as the Humpty-Dumpty effect [43] , [44] , [45] . Here we report, what is to the best of our knowledge, the first observation of spatial interference fringes with a measurable phase stability, originating from spatially separated paths in SG interferometry. We propose and demonstrate a field gradient beam splitter (FGBS) that may be viewed as the application of modern atom optics to the near-century old idea, where we take advantage of the high magnetic field gradients, fast timing and high accuracy made available on an atom chip. Although our method uses the SG effect, it is very different from previous theoretical [42] , [43] , [44] , [45] , [46] and experimental [47] , [48] schemes of SG interferometry. Although previous experiments used thermal atomic beams in which two spin states propagated on a metre scale, our experiment uses ultracold wavepackets on the micrometre scale. This allows not only for miniaturization, but also the accurate manipulation of the quantum state, enabled by the atom chip. Moreover, as we use minimal uncertainty wavepackets, the phase dispersion due to the evolution through the inhomogeneous potential is considerably smaller. Another fundamental difference is that, in contrast to previous SG interferometer schemes, the time scales in which atoms propagate while in a superposition of two different spin states are extremely short, as the output of the beam splitter demonstrated here contains different momentum states of the same spin state, a crucial advantage in noisy environments. This is why, in contrast to previous experiments, our experiment does not require magnetic shielding. In an operation time of just a few μs, the FGBS may allow for a continuous range of momentum splitting of over 100 photon recoils (100 ħk , for reference photons of 2 π / k =1 μm wavelength). This may enable the advantageous large-angle interferometers [49] , [50] , [51] , [52] , giving rise to highly sensitive probes. As a novel method that combines high momentum splitting with the advantages of chip-scale integration, the FGBS may serve for exploring new regimes of fundamental studies and technological applications. General splitting scheme The general scheme of the FGBS and its output is demonstrated in Fig. 1a–f . It is based on a combined manipulation of two internal states (|1› and |2›) and an external potential. We perform a Ramsey-like sequence of two π/2 Rabi rotations and apply a field gradient during the time interval between them. The states |1› and |2› may be any two states enabling controlled coherent transitions between them, and having a state-dependent interaction with the field gradient. We start with the atoms in the internal state |2› and an external state | p 0 , x 0 ›, representing a wavepacket with central momentum p 0 and central position x 0 . The first π/2 rotation transfers the atoms into the superposition state . We then apply a field gradient that constitutes a state-selective force F j =− V j ( j =1, 2) for an interaction time T , which is typically shorter than the time it takes the atoms to move in the force field. The state of the atoms after time T is then , where each level acquires a phase gradient [− V j ( x ) T / ħ ]= F j T / ħ , which is equivalent to a momentum transfer p 0 → p 0 + F j T . 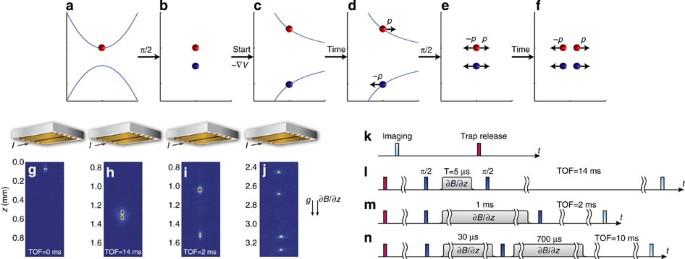Figure 1: The FGBS at work. (a–f) General operation scheme. (a) Atoms in the state |2› (red) are released from a trap. (b) A π/2 pulse splits the wave-function into a superposition of internal levels |1› (blue) and |2›. (c) A state-dependent force is applied. (d) Atoms in the two internal states are accelerated into different momenta. (e) The force is turned off and another π/2 pulse produces a superposition of four parts with two different momenta and two different internal states. (f) After some evolution time, the momentum components are split spatially. (g–j) FGBS input–output images: (g) In the trap before the release. (h) After a weak splitting of less thanħkusing 5 μs of interaction time and allowing for 14 ms TOF. (i) After a strong splitting of more than 40ħkusing 1 ms interaction time and allowing for 2 ms TOF. (j) To view all four output wavepackets predicted by equation (1), we separate the two internal states by another strong gradient pulse. Imageshandishow the large dynamic range this method makes available without any complicated sequence. (k–n) Schematic descriptions of the experiments shown in imagesg–j, respectively. The chip is produced at the Ben–Gurion University fabrication facility. The second π/2 rotation transfers the atoms into the superposition state Figure 1: The FGBS at work. ( a – f ) General operation scheme. ( a ) Atoms in the state |2› (red) are released from a trap. ( b ) A π/2 pulse splits the wave-function into a superposition of internal levels |1› (blue) and |2›. ( c ) A state-dependent force is applied. ( d ) Atoms in the two internal states are accelerated into different momenta. ( e ) The force is turned off and another π/2 pulse produces a superposition of four parts with two different momenta and two different internal states. ( f ) After some evolution time, the momentum components are split spatially. ( g – j ) FGBS input–output images: ( g ) In the trap before the release. ( h ) After a weak splitting of less than ħk using 5 μs of interaction time and allowing for 14 ms TOF. ( i ) After a strong splitting of more than 40 ħk using 1 ms interaction time and allowing for 2 ms TOF. ( j ) To view all four output wavepackets predicted by equation (1), we separate the two internal states by another strong gradient pulse. Images h and i show the large dynamic range this method makes available without any complicated sequence. ( k – n ) Schematic descriptions of the experiments shown in images g – j , respectively. The chip is produced at the Ben–Gurion University fabrication facility. Full size image representing two wavepackets with momenta p j = p 0 + F j T entangled with the internal states , such that each of the internal states |1› and |2› is in a superposition of wavepackets with different momenta (the state in equation (1) can be viewed as spatial Ramsey fringes, see below). Equation (1) is also valid if the atomic motion during the interaction time is taken into account or when the force is not homogeneous in space and time. In this case, the states | p j , x 0 › should be replaced with the more general solutions for the wavepacket evolution in the respective potentials V j ( x , t ). This completes the operation of momentum splitting. One may then use the |1› and |2› states to realize two parallel interferometers for noise rejection. One can also use the entangled momentum and internal state as an interferometer of two clocks (for example, ref. 53 ). If one wishes to stay with just one of the two internal states, one may typically find a dedicated transition to discard the redundant state. Realization of the FGBS To realize the FGBS, we use Zeeman sublevels of freely falling 87 Rb atoms and magnetic field gradients from a chip wire. We start with a BEC of ~10 4 atoms in state | F , m F ›=|2, 2› ≡ |2› and use a RF field to perform transitions to state |2, 1› ≡ |1›. We use the same setup described in ref. 54 . The trap position is at a distance of z =100 μm from the chip surface, and the radial and axial trapping frequencies of |2› are ≈2 π × 100 Hz (measured) and ≈2 π × 40 Hz (estimated), respectively. In order to have the |1› and |2› states form a pure two-level system, we apply a strong homogeneous magnetic field (Δ E 12 ≈ h × 25 MHz) and push the transition to |2, 0› out of resonance by ~250 kHz due to the non-linear Zeeman effect [54] . Next, we release the BEC and apply two π/2 RF pulses with a Rabi frequency of Ω R =20–25 kHz and with a magnetic gradient pulse of length T in between, thus forming a Ramsey-like sequence. The gradient is generated by a current of 2–3 A in a 200 × 2 μm 2 gold wire on the chip surface. The homogeneous magnetic field (in the direction of the magnetic field generated by the chip wire) is kept on during the free fall to preserve the quantization axis. In Fig. 1g–j , we demonstrate the output of the FGBS splitting process. Figure 1g presents an image of the cloud in the trap, before it is released. In Fig. 1h-1i , we present an image of the output of two events that exhibit the large dynamic range of this method, one with momentum difference of less than ħk ( T =5 μs), and the other with more than 40 ħk ( T =1 ms). To compare with atom interferometry based on light beam splitters, we express the momentum transfer in units of ħk , where ħk is a reference momentum of a photon with 1 μm wavelength. The only parameter that is changed is the interaction time T . Finally, in order to verify the internal state of the atoms (equation (1)), we separate between the |1› and |2› states by a second long pulse of magnetic field gradient, as shown in Fig. 1j . 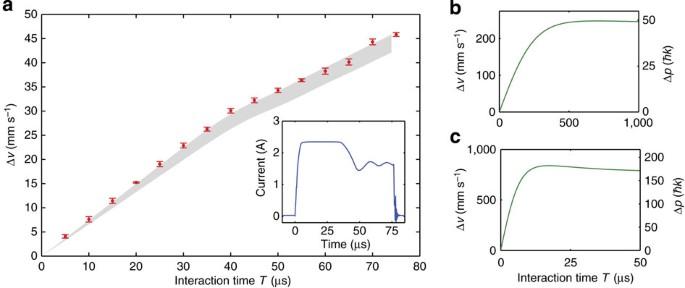Figure 2: Characterization of the FGBS momentum output: (a) The velocity difference between the two observed clouds as a function of the interaction timeT. The error bars are calculated from the variation of a few data sets. The theoretical prediction (shaded area) is based on a measured current in a resistor that mimics the chip wire (inset), taking into account errors of ±2.5 μm (one pixel) in the initial cloud position, ±0.2 Ω in the wire resistance and a 1 μs delay of the measured rise-time (due to the resistor's inductance). The linear dependence onTis to be expected from the solution of equation (2). The current ‘overshoot’ at short times is responsible for the larger acceleration for smallT. (b) Numerical integration of equation (2) overT, using the experimental wire configuration and using a constant current of 3A. We observe the limit of our specific FGBS realization due to the large distance that develops between the atoms and the wire. (c) Using improved experimental parameters, we find that Δpof above 100ħkis possible in less than 10 μs. The parameters are:z=10 μm andI=2A, and the wire dimensions are 10 × 2 μm2(107A cm−2is safely achievable for such short pulses). Figure 2a shows the measured differential momentum transfer as a function of the interaction time T . An interaction time as short as 100 μs is required to transfer a relative velocity of 50 mm s −1 (equivalent to 10 ħk ). The operation of the FGBS may be quantitatively understood by simple kinematics in one dimension (along the z axis). During the interaction time T , a differential acceleration between the wavepackets is induced, such that after the FGBS, each internal state is a superposition of two wavepackets which were accelerated as a |1› or |2› state. The force applied on a wavepacket of a certain m F state at a distance z below the chip wire is: Figure 2: Characterization of the FGBS momentum output: ( a ) The velocity difference between the two observed clouds as a function of the interaction time T . The error bars are calculated from the variation of a few data sets. The theoretical prediction (shaded area) is based on a measured current in a resistor that mimics the chip wire (inset), taking into account errors of ±2.5 μm (one pixel) in the initial cloud position, ±0.2 Ω in the wire resistance and a 1 μs delay of the measured rise-time (due to the resistor's inductance). The linear dependence on T is to be expected from the solution of equation (2). The current ‘overshoot’ at short times is responsible for the larger acceleration for small T . ( b ) Numerical integration of equation (2) over T , using the experimental wire configuration and using a constant current of 3A. We observe the limit of our specific FGBS realization due to the large distance that develops between the atoms and the wire. ( c ) Using improved experimental parameters, we find that Δ p of above 100 ħk is possible in less than 10 μs. The parameters are: z =10 μm and I =2A, and the wire dimensions are 10 × 2 μm 2 (10 7 A cm −2 is safely achievable for such short pulses). Full size image where μ 0 and μ B are the magnetic permeability of free space and the Bohr magneton, g F is the Landé factor for the hyperfine state F and I is the current. The equation does not include the effect of nonlinear Zeeman splitting and a geometric term 1/[1+( W /2 z ) 2 ], accounting for the finite width W of the wire. These terms have been taken into account in our full simulation of the FGBS which, as presented in the figure, is in good agreement with the experimental results. The linear relation in Fig. 2a is to be expected for the short interaction times during which the atoms move only slightly, and the acceleration in equation (2) is fairly constant (the kink in Fig. 2a is due to changing currents, see caption). In Fig. 2b , we present the calculated limit of our specific realization of the FGBS because of the growing distance of the atoms from the gradient source, the chip wire. In Fig. 2c , we show that for realizable chip wire parameters, momentum transfers of over 100 ħk are feasible in a few microseconds. The FGBS output as a spatial Ramsey fringe pattern In Fig. 3 , we present a Gross–Pitaevskii simulation of the atomic density for state |2› just after the second π/2 pulse (‘near field’). The density shows a sinusoidal pattern. This pattern may be viewed as spatial Ramsey fringes: an atom at a specific point x is subjected to a Ramsey sequence in which the phase accumulated between the two π/2 pulses is (1/ ħ ) where Δ V = V 1 − V 2 is the potential difference between the two levels. As the potential approximately varies linearly along the axis, Δ V ≈−Δ Fz , and at short times the atom stays stationary, the Ramsey phase and consequently the population of the two states |1› and |2› is modulated with a wavelength λ = h /2Δ FT (where the factor 2 is due to the fact that we observe intensity modulations and not amplitude). As a perfect sine function Fourier transforms into two identical and counter propagating k components (with momentum difference Δ p = h /2λ), this ‘near-field’ density distribution transforms after a sufficient time-of-flight (TOF) into a pair of spatially separated wavepackets. The ‘near-field’ fringes shown in the figure are not resolvable by our imaging system, and what we observe is only the four wavepackets (two for the state |1› and two for the state |2›) that evolve after a long TOF, as shown in Fig. 1 . 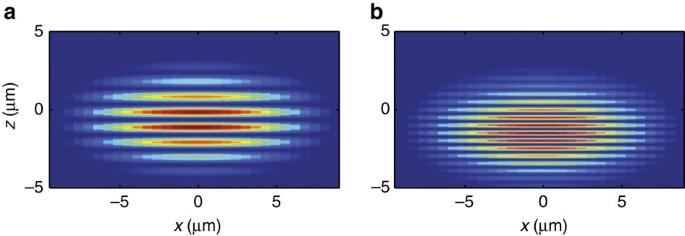Figure 3: Simulation of the splitting process (Gross–Pitaevskii): For interaction times, (a)T=5 μs and (b)T=10 μs, we present the atomic density for state |2› of the ‘near-field’ fringes formed just after the FGBS (no TOF). The sine function Fourier transforms into two counter propagating momentum components, which may be observed as two separated wavepackets after sufficient TOF. Figure 3: Simulation of the splitting process (Gross–Pitaevskii): For interaction times, ( a ) T =5 μs and ( b ) T =10 μs, we present the atomic density for state |2› of the ‘near-field’ fringes formed just after the FGBS (no TOF). The sine function Fourier transforms into two counter propagating momentum components, which may be observed as two separated wavepackets after sufficient TOF. Full size image Observation of interference In order to examine the coherence of the FGBS output, we have applied a simple procedure to stop the relative motion of the two output wavepackets of internal state |2›. We then let them freely expand and overlap to create spatial interference fringes, as shown in Fig. 4 (the state is out of the field of view). This method is suitable for the observation of interference between wavepackets with small spatial separation. If the spatial separation and the momentum difference is large, the wavelength of the interference pattern may be smaller than the resolution limit of the imaging system. In this case, interferometric methods based on internal state population should be applied (see Discussion). 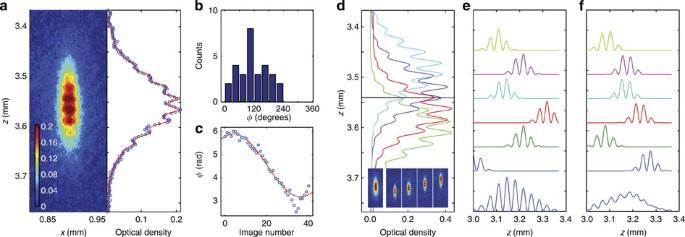Figure 4: Phase stability analysis: (a) Averaged optical density image of a set of 29 consecutive single images in the first half hour of an interferometric measurement session (one image per minute), and a one-dimensional cut (data and fit, see text). The visibility of the averaged fringe pattern reduces to 0.09±0.01, relative to the single-shot value of 0.20±0.02. The average wavelength is similar, 23.1±0.35 μm in the single shots and 22.9±0.2 μm in the averaged image. (b) Phase distribution of the 29 images in π/6 radian bins, with a width of 1.04 radians (r.m.s.), in accordance with that expected by our stability analysis, see text. A random distribution has a probability of 3 × (2/3)29=2.5 × 10−5of similarly occupying only 2/3 of the phase spectrum. (c) Phase of fringes of averaged running sets (‘windows’) of 16 images over a total set of 55 consecutive images. This shows a long-term variation of the phase that is approximated by a sine fit (solid line) with an amplitude of 1.35 radian and a period of 65 min. The 29 images analysed inawere taken near the maximum of the long-term variation. (d) Sample of four fits of single images, demonstrating the small variation of the fringe phase with respect to a fixed position, while the envelope of the pattern changes with no correlation to the fringes. The images from which the fits were taken are also shown, together with the averaged image ofa. (e,f) Gaussian wavepacket model (see text) of interference pattern stability for parameters similar to those used in the experiment (neglecting atom–atom interactions). The six upper plots demonstrate single-interference events, where the interference patterns appear at different positions due to momentum fluctuations caused by an instabilityδzi=1 μm in the initial wavepacket position. Ine, the chip wire current fluctuations are assumed to beδI/I=10−6. Phase instability is negligible and the averaged interference pattern (over 100 single patterns) is almost perfect (bottom plot). Inf, same asewithδI/I=10−3. Phase fluctuations are aboutδ~1. radian and the visibility of the average pattern is low. Figure 4: Phase stability analysis: ( a ) Averaged optical density image of a set of 29 consecutive single images in the first half hour of an interferometric measurement session (one image per minute), and a one-dimensional cut (data and fit, see text). The visibility of the averaged fringe pattern reduces to 0.09±0.01, relative to the single-shot value of 0.20±0.02. The average wavelength is similar, 23.1±0.35 μm in the single shots and 22.9±0.2 μm in the averaged image. ( b ) Phase distribution of the 29 images in π/6 radian bins, with a width of 1.04 radians (r.m.s. ), in accordance with that expected by our stability analysis, see text. A random distribution has a probability of 3 × (2/3) 29 =2.5 × 10 −5 of similarly occupying only 2/3 of the phase spectrum. ( c ) Phase of fringes of averaged running sets (‘windows’) of 16 images over a total set of 55 consecutive images. This shows a long-term variation of the phase that is approximated by a sine fit (solid line) with an amplitude of 1.35 radian and a period of 65 min. The 29 images analysed in a were taken near the maximum of the long-term variation. ( d ) Sample of four fits of single images, demonstrating the small variation of the fringe phase with respect to a fixed position, while the envelope of the pattern changes with no correlation to the fringes. The images from which the fits were taken are also shown, together with the averaged image of a . ( e , f ) Gaussian wavepacket model (see text) of interference pattern stability for parameters similar to those used in the experiment (neglecting atom–atom interactions). The six upper plots demonstrate single-interference events, where the interference patterns appear at different positions due to momentum fluctuations caused by an instability δz i =1 μm in the initial wavepacket position. In e , the chip wire current fluctuations are assumed to be δI/I= 10 −6 . Phase instability is negligible and the averaged interference pattern (over 100 single patterns) is almost perfect (bottom plot). In f , same as e with δI/I =10 −3 . Phase fluctuations are about δ ~1. radian and the visibility of the average pattern is low. Full size image The simple procedure we use to stop the relative motion consists of applying a second gradient pulse giving a stronger kick to the wavepacket with smaller momentum, which is at this time closer to the chip wire relative to the wavepacket with larger momentum. The duration of the second momentum kick is tuned such that after this kick the two wavepackets have the same momentum (with a spatial separation that we denote by 2 d ). In order to understand the formation of the interference pattern, we use a Gaussian model in which the two interfering state |2› wavepackets | p 1 , z 1 › and | p 2 , z 2 › have a Gaussian shape of initial width σ 0 and centre trajectories z 1 ( t ) and z 2 ( t ), corresponding to atoms that have been in the internal states |1› and |2›, respectively, during the FGBS gradient pulse (see Methods for more details). Given that the final momentum difference between the two interfering wavepackets is smaller than the momentum spread of each one of them, after a long enough time they overlap and an interference pattern appears having the approximate form: where A is a constant, z CM =( z 1 + z 2 )/2 is the centre-of-mass (CM) position of the combined wavepacket at the time of imaging, σ z ( t ) ≈ ħt /2 mσ 0 is the final Gaussian width, λ = ht /2 md is the fringe periodicity (2 d =| z 1 − z 2 |), v is the visibility and φ = φ 2 − φ 1 is the global phase difference. The phases φ 1 and φ 2 are determined by an integral over the trajectories of the two wavepacket centres. We emphasize that equation (3) is not a phenomenological equation, but rather an outcome of our analytical model (see Methods ). Equation (3) is used for fitting the interference patterns as those shown in Fig. 4 . For a pure superposition state, as in our model, the fringe visibility v should be 1. The observed visibility is reduced because of various possible effects, such as unequal amplitudes of the two wavepackets or partial overlap between them, the finite temperature of the atomic cloud, effects of atomic collisions and limited imaging resolution. We note that some of the many-body collisional effects, such as phase diffusion, would not lead to a reduction of the single-shot visibility, but may cause the randomization of shot-to-shot phase. As the single-shot visibility does not imply that the interferometric process is coherent, one needs to examine the stability of the phase along many experimental realizations of the interference. Phase and momentum stability An analysis of a sequence of interference patterns ( Fig. 4a–c ) reveals short-term phase fluctuations of δφ ~1 radians and long-term drifts over a time scale of an hour. The coherence of the underlying interferometric process is clearly proven by this analysis. In particular, we directly observe statistically significant phase repeatability in a time window of about half an hour where the drift is slow, such that an image obtained by averaging over the 29 single-shot images shows a pronounced visibility of only a factor of ~2 less than the single-shot visibility. To identify the sources of instability and to suggest ways to reduce it, we analyse the propagation of the wavepackets with the help of our Gaussian model. This analysis shows that the major source of phase instability in our experiment is the difference in magnetic field energy during the time between the two π/2 pulses of the FGBS, in which the two wavepackets occupy two different spin states. As the magnetic energy is linearly proportional to the pulse current, the phase fluctuation at a given reference point z 0 is where the relative current fluctuations during the pulse δI / I and the timing uncertainty δT / T are both independently estimated for our electronics to have a root-mean-square (r.m.s.) value of ~10 −3 . As the field applied by the chip wire at z 0 =100 μm is about 27 G, corresponding to a Zeeman potential of ~19 MHz, we expect, for T =5 μs, phase fluctuations of δφ ~1 radian, similar to the observed short-term phase fluctuations (width of the phase distribution in Fig. 4b ). Note that during the 100 μs time interval between the two π/2 pulses, a bias field of about 40 G (in the same direction as the wire field) is on. Changes in the distant coils responsible for this field are most likely the source of the observed long-term drift of the phase. Although the FGBS intrinsic phase instability was found to be the main source of the interferometric phase instability in our experiment, it is important to analyse the FGBS momentum instability, which may become the dominant factor in interferometers with a larger space-time area. In Fig. 4d , we show a few images and fits of single-interference patterns that reveal an instability in the CM momentum. The source of this instability may be understood on the basis of equation (2), indicating that the momentum kick fluctuations of our FGBS are given by where z i is the initial distance from the wire responsible for the momentum kick. As the trapping potential was generated by a wire at a distance of more than 1 mm (with its own relative current fluctuations δI / I ~10 −3 ) rather than a chip wire (for technical reasons), we estimate the uncertainty of this position to be δz i ~1 mm × 10 −3 =1 μm. For z i =100 μm, we have δz i / z i ~10 −2 , making it the dominant source of momentum instability. Indeed, the observed width of the final CM position distribution is δz CM / z CM ~0.02. However, perhaps surprisingly, the observed momentum difference between the two wavepackets after the second momentum kick is much more stable and gives rise to a good overlap at each experimental shot, as observed in Fig. 4 . Let us elaborate. We have approximated the 1/ z potential in our experiment by a quadratic form where represents the inhomogeneity of the force =− ( z , t )/ ∂z , acting as a harmonic force when <0. The observed stability, namely the small relative momentum fluctuations, is due to the fact that the second momentum pulse reverses the effect of momentum fluctuations due to the first pulse. The second pulse applies a differential force F 2 ( z 1 )− F 2 ( z 2 )= F ′ 2 ( z 0 )( z 1 − z 2 ) ∝ −( p 1 − p 2 ), which acts against initial momentum fluctuations. In the interferometric scheme used in our experiment, the second pulse introduces its own fluctuations of the momentum difference through current fluctuations δI and δT , but as noted, this contribution is an order of magnitude smaller than that of the fluctuations introduced by the initial position fluctuations during the first pulse. Finally, our Gaussian model shows that initial position fluctuations contribute very little to the fluctuations of the accumulated phase difference after a long TOF. As demonstrated in Fig. 4e , initial position fluctuations give rise to fringe patterns whose Gaussian envelopes appear at a different position in each shot, but their phase is the same in the lab frame. This decoupling between the wavepacket position and its phase is also observed in the experiment, as demonstrated in Fig. 4d . Significant phase fluctuations that reduce the visibility of the averaged pattern are mainly caused by current strength and timing fluctuations during the gradient pulse ( Fig. 4f ), as discussed above. Here we have used the old idea of SG interferometry as a basis for a novel method in atom chip interferometry, and observed stable interference fringes from spatially separated paths. This achievement is due to three main differences compared with previous SG schemes. First, the use of minimal uncertainty wavepackets (a BEC) rather than thermal beams. Second, in most of the interferometric cycle, the two interferometer arms are in the same spin state. Finally, chip-scale temporal and spatial control allows the cancellation of path difference fluctuations. The FGBS has two main advantages in comparison to previously demonstrated matter-wave beam splitters: its tuneable high dynamic range of momentum transfer and its natural integrability with an atom chip. Compared with previous atom chip experiments with double-well potentials, which are limited to relatively slow splitting to prevent higher mode excitations, the FGBS allows a wide range of splitting times that will enable the investigation of many-body effects of entanglement and squeezing over new parameter regimes. For example, in the presence of atom–atom interactions, generation of a coherent many-body state is possible only by fast splitting [28] . On the other hand, the FGBS that uses magnetic field gradients for splitting is more naturally and easily suited for integration with an atom chip compared with laser light splitting methods. These advantages are expected to make FGBS-based interferometry suitable for high sensitivity measurements on the micron scale. We have gained an accurate understanding of the sources of instability in our experimental system that was not dedicated to atom interferometry, and used a simple wire configuration as well as electronics with significant technical noise. We have shown that our Gaussian model correctly predicts the position and phase fluctuations of the observed fringes, as well as the decoupling between the position and phase. We may thus attempt to suggest prospects for the stability in future experiments. A straight forward way to improve phase stability (equation (4)) is to improve the stability of current amplitude and timing. In addition, one can use a configuration with decreased ratio between the magnetic field at the trapping position and its gradient (see equation (2)), such that the momentum kick may be increased while keeping the same phase fluctuations, or the phase fluctuations may be reduced while keeping the same momentum kick. One way to achieve this is to set the initial trapping position z 0 closer to a narrower chip wire. An alternative way is to use three parallel wires with alternating currents, such that a quadrupole field is formed near the initial position of the atoms. Such a field provides a high gradient and a small absolute value of the magnetic field. Momentum kick variations may also be reduced by using chip-based initial trapping for a better control of the initial position. In order to estimate the bounds on phase and momentum stability in future realizations, one should consider the available technology. Let us assume a 10-μs pulse. Then, for a 2A current (containing ~10 14 electrons), the shot noise leads to δ ( IT )/ IT ~10 −7 . Power sources with sub-shot noise are being developed (for example, at Jet Propulsion Laboratory [55] ) and may enable an even better stability. Stable current pulses may be driven by ultra stable capacitors, which reach stability of δC / C =10 −7 at mK temperature stabilities. For pico-second switching electronics, one similarly finds δT / T ~10 −7 . Taking these limits and assuming that the momentum pulse could be performed in a medium magnetic field of 1 G (splitting of 0.7 MHz), the limit on the phase uncertainty of the FGBS becomes δφ ~6 × 10 −6 radian, while momentum stability is bound by δp / p ~10 −7 . Phase and momentum stability may improve even more for longer and larger current pulses giving rise to higher momentum transfer, as the relative timing instability and shot noise reduces. A more careful estimation would require taking into account the specific structure of the FGBS and the whole interferometer, as well as environmental factors such as thermal expansion of chip elements. As an outlook for guided interferometry, an alternative scheme using trapped atoms was implemented, though currently without fringe repeatability (S.M., Y.J., R.F., manuscript in preparation). Other possible alternatives for the operation of the FGBS include different level schemes. One example is the possible use of magnetically insensitive atomic levels such as |2, 0›. A superposition of two momentum states of |2, 0› can be easily achieved by a Rabi rotation with a RF pulse tuned to the transition |2, 1› →|2, 0›. Another example is a FGBS using a microwave transition between two hyperfine states with opposite magnetic moments, such as the states |2, 1› and |1, 1›, enabling symmetric splitting with opposite momenta. Through nonlinear Zeeman effect, the FGBS may also split directly the magnetic noise immune ‘clock’ states |1, 0› and |2, 0› (see Methods ). Finally, we propose two interferometer schemes, each based on two FGBSs. The first scheme creates spatial fringes and replaces the second momentum kick used in our experiment with a second FGBS when the spatial separation between the two wavepackets is 2 d , as described in Fig. 5a–c . Unlike the method used in the current experiment, which is based on a long inhomogeneous gradient pulse, the proposed method uses a short pulse with the price of reducing the signal intensity by a factor of 2. The second scheme realizes internal state population fringes and requires reversing the velocity of the wavepackets. When the two parts of the wave-function spatially overlap, another FGBS is applied, as described in Fig. 5d–f . See Methods for more details. In view of the versatility of the FGBS, we expect it to enable a wide range of fundamental as well as technological applications. 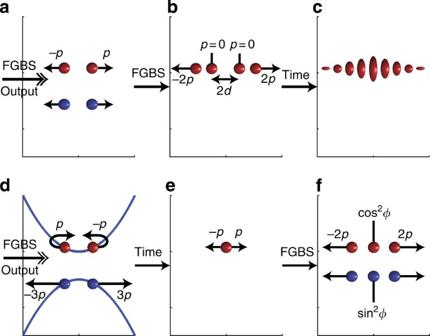Figure 5: Alternative schemes for FGBS-based interferometry. (a–c) Spatial signal interferometer. (a) After the FGBS, the two momentum components are split spatially. (b) Another FGBS is applied, creating four clouds (considering only the |2› state). Two are at rest and two are at ±2p. (c) After some evolution time, the two clouds that are at rest expand, overlap and create a spatial interference pattern. (d–f) Internal state signal interferometer. (d) After splitting and propagation, a returning force is applied for state |2›, which reverses the motion of state |2› and repels state |2›. (e) After an evolution time, the two momentum components overlap in space. (f) A second FGBS is applied, forming a superposition of three momentum components, such that the internal state population of the middle component depends on the relative phase between the two parts of the wave-function just before the second FGBS. Figure 5: Alternative schemes for FGBS-based interferometry. ( a – c ) Spatial signal interferometer. ( a ) After the FGBS, the two momentum components are split spatially. ( b ) Another FGBS is applied, creating four clouds (considering only the |2› state). Two are at rest and two are at ±2 p . ( c ) After some evolution time, the two clouds that are at rest expand, overlap and create a spatial interference pattern. ( d – f ) Internal state signal interferometer. ( d ) After splitting and propagation, a returning force is applied for state |2›, which reverses the motion of state |2› and repels state |2›. ( e ) After an evolution time, the two momentum components overlap in space. ( f ) A second FGBS is applied, forming a superposition of three momentum components, such that the internal state population of the middle component depends on the relative phase between the two parts of the wave-function just before the second FGBS. Full size image To conclude, we have demonstrated a method for splitting atoms into momentum states by using local magnetic field gradients and have observed repeatable spatial interference fringes, which indicate the coherence of the splitting process. The method has a wide dynamic range of momentum transfer, it is versatile in geometry and utilized states, and is easily integrable with an atom chip. We have analysed in detail the causes for phase and momentum instabilities. Our analysis exhibits a good fit to the experimental observations. Based on this analysis, we propose practical ways to exploit the potential of the wide dynamic range of momentum transfer and to increase interferometric stability. This enables us to extrapolate and predict the ultimate accuracy of such a device—which we find to be high. Gaussian wavepacket model for interferometry Our model assumes that the atomic state at each stage of the interferometric process is a superposition of wavepackets as in equation (1). The spatial representation can generally be written as where | w j › represent internal state trajectories, such that at time t , two states | w j › and | w k › may either represent two different internal states or the same internal atomic state with different internal state histories. In our case, for example, the state | w 1 › will represent atoms that were initially at the state | m F =2›, then transformed into | m F =1› during the first π/2 pulse and then back to | m F =2› during the second π/2 pulse, and | w 2 › will represent a trajectory where the atoms stayed at | m F =2› throughout this process. In what follows, we omit the ket symbols | w j › whenever they represent the same internal state at time t . In equation (7), ψ j ( z , t ) represent spatial wave-functions that we take as Gaussian wavepackets where a j , b j and c j are complex. This is equivalent to the form where Z j ( t ) is the central position and P j ( t ) is the central momentum of the j 'th wavepacket, whereas φ j is a real phase of the wavepacket at the centre. We assume that the potential is smooth enough on the scale of the wavepacket, such that it can be approximated by a quadratic form as in equation (6) with the force F j =−∂ z V j and the potential curvature (with m F → j ). With this approximation and neglecting atom–atom interactions, the Gaussian ansatz is an exact solution for the propagation problem. By substituting the Gaussian form (8) in the Schrödinger equation and equating terms proportional to z 2 , z and 1, we obtain the equations for the coefficients By comparing the forms (8) and (9) we find b j =2 a j Z j + iP j / ħ and , where the equations for the centre coordinates are given by the Newtonian equations of motion where the solution for the phase in the wavepacket CM frame is An analytical solution for a j is possible for constant coefficients F j and F ′ j where with and Let us now take a superposition of two wavepackets of the form (9) with equal amplitudes C j and widths ( a 1 = a 2 = a ). We obtain where Z CM =( Z 1 + Z 2 )/2 is the position of the CM of the two wavepackets and P CM =( P 1 + P 2 )/2 is the CM momentum, whereas Δ z = Z 1 − Z 2 and Δ p = P 1 − P 2 are the corresponding position and momentum differences. ψ CM ( z ) is the wave-function of the form of equation (9) with Z CM , P CM and φ CM ≡( φ 1 + φ 2 )/2 replacing the corresponding single-wavepacket coordinates and phase. The exponential arguments are In free-space propagation we have a ( t )= a (0)(1+2 ia (0) ħt / m ) −1 . By substituting Z j ( t )= Z j (0)+ P j t / m in the expression for ξ j we obtain After a time t , such that t m /2 ħ | a (0)|, we have a ( t )~− im /2 ħt such that the term containing the momentum vanishes. The atomic density per unit length is given by N | ψ ( z )| 2 , where N is the total atom number. In the long time limit, the coefficient a becomes imaginary, such that ξ j and θ j in equation (17) become imaginary as well. The last line of equation (17) becomes cos(Δ ξz +Δ θ /2)=cos( m d z / ħt + φ /2), where 2 d = Z 2 − Z 1 and φ = θ 2 − θ 1 . To obtain equation (3), we take the square absolute value of equation (17), and use Re{ a ( t )}=1/4 σ z ( t ) 2 and . The visibility v is ideally equal to 1 and was included as a parameter in equation (3) in order to account for the real interference patterns whose visibility is lower than the ideal one. Splitting magnetically insensitive states Another interferometric scheme that is based on the same idea of the FGBS involves the two first-order magnetically insensitive substates |1,0› and |2,0› of the two hyperfine states, which are analogous to those used in present-day precision interferometers. A microwave π/2 pulse may be used to create an equally populated superposition of the two states and then they may be split into two momentum states using a magnetic gradient at a high magnetic field. The non-linear Zeeman shift of the transition energy between the states is Δ E ≈ α B 2 , where α =2 πħ × 575 Hz G −2 . At a distance of 10 μm from a wire carrying 2A of current, the atoms are exposed to a magnetic field of B =400 G and a magnetic gradient of ∂ z B =40 kG mm −1 . It then follows that F = ∂ z Δ E ( z )=2 πħ × 575 × 2 B∂ z B =1.22 × 10 −20 N, and consequently atoms receive a differential velocity of 84.7 mm s −1 for a 1-μs pulse, equivalent to about 18 ħk . As the two states are relatively magnetically insensitive, the second π/2 pulse of the FGBS would not be needed and the two output beams of this beam splitter could be used for interferometry in a completely analogous way to existing interferometers based on light beam splitters. Recombining the two wavepackets similarly requires only a gradient and one π/2 pulse, and the internal state population can now be measured. Future interferometry schemes In order to construct a full interferometer based on spatial or internal state interference, one needs to recombine the two momentum outputs of the FGBS. Here we present two schemes to recombine the two momentum outputs of the FGBS and create a full interferometer, with spatial or internal state interference signals. In the CM frame, an atom that was accelerated by the force F 2 ( F 1 ) is at time t after the FGBS in the state | p , d › (|− p ,− d ›) where p =( p 2 − p 1 )/2 and d = p t / m represent the external degrees of freedom of the centre of the wavepackets, m being the mass. At this point, their relative motion can be stopped and after sufficient free expansion time (or TOF) t TOF they overlap and create a spatial fringe pattern with periodicity λ = ht TOF /2 md . The simplest way to stop the relative wavepacket motion is to apply a gradient (for example, an harmonic potential), which will accelerate each part of the wave-function in an opposite direction. This method was followed in our experiment, as described in the text. Another way to stop the relative motion of the two wavepackets is to apply the FGBS again, as shown in Fig. 5a–c . Considering only the state |2›, the spatial wave-function in the CM momentum and position coordinates is , where φ is the relative phase accumulated between the two paths during the propagation. After the second FGBS, which applies a momentum difference p ′, the new wave-function in the CM frame is such that if p ′=± p we are left with two wavepackets with the same momentum at ± d , giving rise to spatial interference after expansion. If one wishes to use the internal state population as a signal, one needs to overlap the two parts of the wave-function spatially and then apply another FGBS, as shown in Fig. 5d–f . Once the wavepackets overlap, the second FGBS is operated, giving rise to a wave-function of the same form as in equation (20) with d →0. If the magnitude of the momentum kick p ′ of the second FGBS is equal to that of the first FGBS, we are left with two wavepackets with a zero CM momentum in an internal state which depends on the propagation phase φ . For p ′= ± p in equation (20), the internal state with zero CM momentum is How to cite this article: Machluf, S. et al . Coherent Stern–Gerlach momentum splitting on an atom chip. Nat. Commun. 4:2424 doi: 10.1038/ncomms3424 (2013).